Molecular solar thermal energy storage in photoswitch oligomers increases energy densities and storage times Molecular photoswitches can be used for solar thermal energy storage by photoisomerization into high-energy, meta-stable isomers; we present a molecular design strategy leading to photoswitches with high energy densities and long storage times. High measured energy densities of up to 559 kJ kg −1 (155 Wh kg −1 ), long storage lifetimes up to 48.5 days, and high quantum yields of conversion of up to 94% per subunit are demonstrated in norbornadiene/quadricyclane ( NBD/QC ) photo-/thermoswitch couples incorporated into dimeric and trimeric structures. By changing the linker unit between the NBD units, we can at the same time fine-tune light-harvesting and energy densities of the dimers and trimers so that they exceed those of their monomeric analogs. These new oligomers thereby meet several of the criteria to be met for an optimum molecule to ultimately enter actual devices being able to undergo closed cycles of solar light-harvesting, energy storage, and heat release. Solar energy is a viable and inexhaustible source of energy for both electricity and heat production. In this context energy storage is a major challenge due to strong daily and seasonal variations in the availability of sunlight [1] . Molecular solar thermal (MOST) systems represent a promising avenue for harvesting and storing solar energy. In this approach a molecule is converted by photoisomerization into a higher-energy isomer, which is capable of storing the energy until released by a heat trigger or catalyst, converting the meta-stable isomer to the original light-harvesting isomer [2] , [3] , [4] , [5] , [6] , [7] , [8] , [9] , [10] . Norbornadienes have shown to be a promising candidate for MOST due to the high energy difference between the norbornadiene ( NBD ) and quadricyclane ( QC ) photoisomer of approximately 96 kJ mol −1 (Fig. 1 ), and the system has been shown to undergo heat-release by the action of cobalt-based catalysts [11] , [12] , [13] . For these systems it has been previously shown that donor–acceptor substitutions provide an effective means for red-shifting the longest-wavelength absorption, improving the solar spectrum match; compounds 1 and 2 present examples of such derivatives [14] . Fig. 1 Molecular system. The norbornadiene ( NBD )–quadricyclane ( QC ) couple and the previously reported monomeric norbornadienes 1 and 2 Full size image Two crucial challenges for a useful MOST system are the achievement of a sufficiently high energy storage density, ideally higher than 300 kJ kg −1 and light-harvesting in the visible region [15] . Functionalization of the norbornadiene with donor and acceptor units has been used to tune absorption maxima, but this positive effect on solar absorption is counter-balanced by higher molecular weights, and hence lower energy densities [11] , [16] . Moreover, the positive effect on solar absorption typically also has a detrimental effect on the energy storage time, which is lowered when absorption is redshifted [14] . One possible solution to overcome this anti-correlation between redshifting and energy density that we present here is to couple one chromophore unit to several photoswitches. Here, in the context of NBD / QC systems, we find that it is attractive to form dimers or trimers, where the NBD units share the same donor and/or acceptor. Previously dimers of photoswitches such as dihydroazulenes [17] , dithienylethenes [18] , [19] , azobenzenes [20] , [21] , and spiropyranes [22] , [23] have been reported. Even other norbornadiene dimers, linked via phthalatamide bonds or conjugated ketones, have been prepared and studied, but showed very low quantum yields [24] , [25] . The idea for the present work was to engineer the stability of the high energy photoisomer by having two electronically coupled photoswitches with separate barriers for thermal conversion (Fig. 2 ). The reasoning for this is that there is a blue shift after the first isomerisation ( NBD–NBD to QC−NBD ), leading to a higher energy of isomerisation of the second switching event ( QC−NBD to QC−QC ). Simultaneously having a shared donor reduces the molecular weight per norbornadiene unit. We chose to synthesize two series of dimers as well as one trimer of NBD that resemble the previously synthesized donor−acceptor monomers 1 and 2 , with absorption onsets of 358 and 374 nm, respectively [14] . Fig. 2 Energy diagram. Schematic representation of the difference in half-life and irradiation energy for the two switching events Full size image Synthesis The synthesis of NBD dimers and trimers is shown in Fig. 3 (all isolated as mixtures of diastereoisomers; only one of these is shown in each case). It was possible to obtain three alkyne-linked dimers as well as one trimer by Sonogashira couplings using the previously reported 2-chloro-3-cyanonorbornadiene 3 as substrate [14] . The simplest dimer was synthesized by Sonogashira coupling with trimethylsilylacetylene, affording 4 in a yield of 63%. The silyl protecting group was removed with potassium carbonate in THF/MeOH, and the resulting terminal alkyne was subjected to a second Sonogashira coupling with 3 to afford the acetylene-linked NBD dimer 5 in 47% yield. In the second Sonogashira reaction, standard conditions using phosphine ligands did not give any of the wanted products due to instability of the terminal acetylene. Instead, the Pd 2 dba 3 /AsPh 3 catalyst system [26] was used as it improved the reaction rate. Utilizing the same reaction conditions as for the synthesis of 4 with either 1,3- or 1,4-diethynylbenzene ( 6 or 7 ) gave the two NBD dimers 8 and 9 in 39 and 31% yield, respectively. Similarly, with 1,3,5-triethynylbenzene 10 as substrate, a triple Sonogashira coupling furnished 11 in a yield of 24%. Fig. 3 Synthesis of alkyne-linked oligomers. Synthesis of acetylene-linked dimers 5 , 8 , and 9 as well as the trimer 11 Full size image To further investigate the effect of the spacer group, a second series with two NBD units directly linked to a phenylene spacer was synthesized (Fig. 4 ). Initial attempts employed 3 as substrate. Yet, a Suzuki cross-coupling with a double boronic acid did not yield any product (see Supplementary Figs. 6 and 8 for conditions). Instead, it was found that the desired product could easily be obtained from a Diels-Alder reaction between the known [27] para and meta bis(cyanoethynyl)benzenes 12 and 13 , respectively, with cyclopentadiene (under microwave heating) affording the dimers 14 and 15 in yields of 77 and 45%. Fig. 4 Synthesis of phenylene-linked dimers. Synthesis of phenylene-linked norbornadiene dimers 14 and 15 . BHT “butylated hydroxytoluene”, i.e., 2,6-di(tert-butyl)-4-methylphenol; MW microwave heating Full size image Spectroscopy The new norbornadiene compounds were investigated with UV-Vis absorption spectroscopy, and the spectra are shown in Fig. 5 . All of the spectroscopic studies were performed in cyclohexane as this solvent gave a larger spectral window for analysis of the switching events than toluene. As expected there is a large difference in the absorption onset and maxima between the meta and para isomers. The systems that are para substituted ( 5 , 8 , and 14 ) give the highest onset of absorbance, which can be explained by the linear conjugation pathway between the two NBD chromophores, providing a larger conjugated system compared to the meta substituted compounds. The spectra of the meta substituted dimer 9 and the trimer 11 have very similar absorption onsets; yet, the trimer with three NBD units has a higher molar absorptivity. Interestingly the spectra are also similar to that of the corresponding monomer 2 (Fig. 5 ) in regard to longest-wavelength absorbance maxima and onset. This trend is also evident in the molar absorptivity, which for compound 2 is approximately half of the value for 9 . The same trend is seen for compounds 1 and 15 , which have comparable absorption onsets and the longest-wavelength absorption maxima. The molar absorptivity of 15 is more than twice that of 1 . Fig. 5 Optical absorption spectra. a UV−Vis absorption spectra of acetylene-linked norbornadienes. Black line: 2 , blue line: 5 , red line: 8 , red dashed line : 9 , green line: 11 . b UV−Vis absorption spectra of phenylene-linked norbornadienes. Black line: 1 , red line: 14 , red dashed line: 15 . The spectra of monomers 1 and 2 were recorded in toluene Full size image The next objective was to study the switching properties of the new NBD−NBD derivatives. 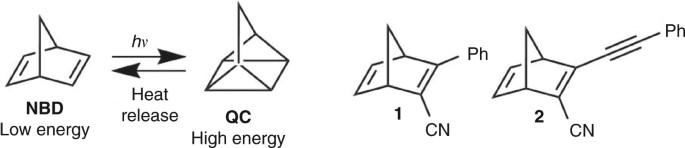Fig. 1 Molecular system. The norbornadiene (NBD)–quadricyclane (QC) couple and the previously reported monomeric norbornadienes1and2 Upon irradiation close to the absorbance maxima (365 or 340 nm), the dimers and trimer could all be fully converted to the corresponding QC−QC dimers, data shown in Table 1 . It was attempted to isomerize all of the norbornadiene dimers selectively to the intermediate QC−NBD form by irradiating around the onset of absorption. Switching to the QC−NBD could be achieved for compounds 5 and 14 by irradiation at 405 nm. In addition the switching events were also studied by NMR spectroscopic analysis. For compound 5 it was found that irradiation at 405 nm forms a thermal-photostationary state between 5 NBD−NBD and 5 QC−NBD , which is dependent on the intensity of the lamp and the temperature of the sample, due to fast back conversion of 5 QC−NBD (vide infra). The ratio found from NMR studies was 54:46 (see Supplementary Fig. 118 ). For 14 , the isomerization to QC−NBD form could be obtained almost quantitatively by irradiation at 405 nm, and the spectra of 14 NBD−NBD , 14 QC−NBD and 14 QC−QC are shown in Fig. 6 . From NMR spectroscopic studies it was found that upon irradiation at 405 nm, small amounts of 14 QC−QC were formed together with 14 QC−NBD , and it was ultimately possible to convert the system to 14 QC−QC although this took over 40 h (see Supplementary Fig. 121 for details). Looking at the absorbance spectrum it is evident that even though it is possible to photoisomerize 14 QC−NBD at 405 nm, the absorbance at 405 nm is close to non-existent, and thereby giving a spectral window for the sequential switching. Table 1 Physical data. Full size table Fig. 6 Stepwise conversion of dimers. a Stepwise isomerization of 5 and 14 to the corresponding QC−NBD and QC−QC isomers. b UV−Vis spectra of 14 and its isomers. Black line: 14 NBD−NBD , blue line: 14 QC−NBD , red line: 14 QC−QC . c UV−Vis spectra of 5 , 5 QC−QC and the thermal-photostationary state between 5 and 5 QC−NBD . Black line: 5 NBD−NBD , blue line: the thermal-photostationary state between 5 and 5 QC−NBD , red line: 5 QC−QC Full size image Quantum yields Quantum yields of the photoisomerization events in cyclohexane were also measured for all the molecules using a reference procedure (Table 1 ) [28] . For some of the molecules, when the absorbance profile allowed it, the quantum yield was measured at different wavelengths. This was done in order to independently probe the quantum yields of the two consecutive photoisomerization processes, ring closure of NBD−NBD and subsequently of QC−NBD (where their absorption profiles were taken into consideration). For compounds 8 , 9 , 11 , and 15 the quantum yields are calculated based on the number of photoconversion events, taking into account that two or three NBD subunits are present per oligomer (see Table 1 ). The assumption is made that the units are behaving like independent NBD units and are having a similar absorption profile. For 14 and 5 , which exhibit sequential switching, it was possible to measure the quantum yield for the NBD−NBD to QC−NBD process selectively. For 5 NBD−NBD it was only possible to measure the quantum yield of the first photoconversion into intermediate 5 QC−NBD due to the fast rate of backreaction. In the case of 14 it is mainly the 14 NBD−NBD form that absorbs, confirmed by the presence of an isosbestic point in the measurement, allowing the formation of 14 QC−QC to be neglected (see Supplementary Fig. 129 ). Furthermore, 14 could be irradiated at 405 nm to form 14 QC−NBD , and subsequently the quantum yield at 340 nm could be measured (see Table 1 ). Kinetics The kinetics of the QC−QC to NBD−NBD backreactions were determined at three different temperatures and the half-life at 25 °C, t ½ (25  °C), was determined from an Arrhenius analysis (Table 1 ). Interestingly, two markedly different rates of back conversion could be measured for both 5 and 14 (see Table 1 ). The half-life for the conversion of QC−NBD to NBD−NBD is remarkably faster than that for the backreaction of the fully isomerized QC–QC isomers. It was possible to fit the data for conversion of 5 QC−QC and 14 QC−QC all the way back to the corresponding NBD−NBD isomers by single-exponential fits, due to the significantly faster conversion of QC−NBD to NBD−NBD . Fascinatingly, the first conversion from QC−QC to QC−NBD exhibits a higher barrier compared to the QC−NBD to NBD−NBD conversion, which we ascribe to the coupled nature of the two different electronic systems. For compounds 8 , 9 , 11 , and 15 a discrimination of the different barriers could not be carried out due to similarities in the electronic properties of the QC−NBD and NBD−NBD forms of the molecules. Cyclability To investigate the stability over several cycles of photoisomerization followed by thermal back-reaction, a cycling test of 8 and 14 was performed (Fig. 7 ) by monitoring the UV−Vis absorption of the compounds at 362 and 350 nm respectively. The cyclability of 8 was tested over 71 cycles at 50 °C giving a decomposition of 0.16% per cycle, and for 14 the decomposition per cycle at 70 °C was found to be 0.11%, showing that the decomposition for both these molecules is very small. This decomposition is shown as a decrease in the absorbance for 8 , while for 14 there is an increase in the absorbance. This increase can be caused by evaporation of the solvent, or a decomposition product with a higher absorptivity. As some evaporation of the solvent could not be avoided, the cyclability of 14 is likely better than observed. Since the backreaction is relatively slow it was not possible to do the experiment at a lower temperature. Fig. 7 Cyclability test. a Cyclability for 8 showing the normalized absorbance at 362 nm in cyclohexane at 50 °C irradiated at 365 nm. 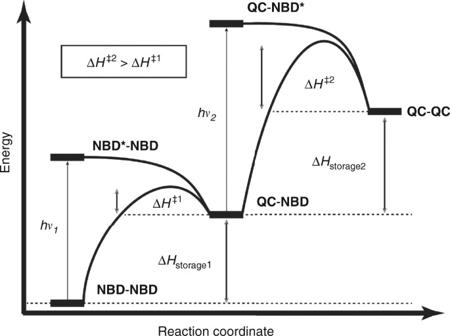Fig. 2 Energy diagram. Schematic representation of the difference in half-life and irradiation energy for the two switching events b Cyclability for 14 showing the normalized absorbance at 350 nm in cyclohexane at 70 °C irradiated at 340 nm Full size image Energy densities To obtain the energy densities of the high-energy QC isomers, the norbornadiene derivatives were irradiated at either 365 or 340 nm in CDCl 3 (CDCl 3 was selected due to the low solubility in cyclohexane), until fully converted; the solutions were concentrated by a stream of nitrogen and the resulting QC subjected to differential scanning calorimetry (DSC) (Table 2 ). Compounds 11 and 14 partly decomposed at the temperatures of the DSC experiment (>140 °C), so the energy densities of these compounds are not included. Isomerization of 5 in either CDCl 3 or toluene- d8 for DSC experiments (~1 M) could not be achieved by irradiation at either 365 or 340 nm, possibly due to lower quantum yields in these solvents as well as the short lifetime of the QC−NBD form (minutes) making quantitative conversions impractical. The heat release data for QC−QC dimers of 8 , 9 , and 15 are listed in Table 2 . For all of the molecules the heat release was also calculated using density functional theory (DFT) calculations (coordinates listed in Supplementary Data) [19] , [20] . The DSC sample for 9 was a mixture of 9 QC−QC and 9 QC−NBD , which results in a large uncertainty, even though a correction taking this into account was performed. This is probably the reason for the large difference between calculated and measured values. Table 2 Energy densities. Full size table In conclusion, we have developed efficient synthetic protocols for the preparation of high-performance norbornadiene dimers and trimers. The quantum yield of photoconversion is near quantitative, up to 94% per NBD subunit. For the para phenylene-bridged NBD dimer 14 , conversions between isomers occurred stepwise—both in the forward and backwards direction—and with significantly different NBD absorption maxima for the NBD−NBD and NBD−QC states. Our molecular design demonstrates the attractive feature of blueshifting the NBD absorption after the first NBD -to- QC photoisomerization as it ultimately furnishes a very energetic QC−QC state after the second photoisomerization as well as a prolonged storage time. As the first energy discharge ( QC−QC to QC−NBD backreaction) is the rate-determining step, full discharge of the system will conveniently be promoted by triggering this event. The system contrasts in this respect related dihydroazulene-vinylheptafulvene dimers incorporated in macrocyclic structures for which instead the first discharge is fast and the second slow [29] . The calculated energy densities of the dimer and trimer systems of up to 927 kJ kg −1 (257 Wh kg −1 ) and measured densities up to 559 kJ kg −1 (155 Wh kg −1 ) greatly exceed the original targets of 300 kJ kg -1 [15] highlighting the potential of applying molecular photoswitches in future solar thermal energy storage technologies. As the strongly coupled dimers 5 and 14 show a higher barrier for the first step in the thermal conversion compared to the second thermal conversion, this molecular motif can be used in future design of high-performance molecular switches for solar thermal energy storage as well as other applications. In future work a donor group could be attached to the benzene ring to give an enhanced redshifting of the absorbance spectra, or changing the benzene ring to more electron-rich aromatics. Another interesting approach would be to have two NBD units directly linked, in an attempt to increase the multimode switching by a greater coupling between the NBD subunits. Materials Cyclopentadiene was distilled by cracking dicyclopentadiene over iron filings and stored at −80 °C, prior to use. Tetrahydrofuran used for Sonogashira coupling reactions was distilled over a sodium/benzophenone couple. All other chemicals were used as purchased from commercial sources. Purification of products was carried out by flash chromatography on silica gel (40–63 μm, 60 Å). Thin-layer chromatography was carried out using aluminum sheets precoated with silica gel. Measurements Infrared (IR) spectra recorded on a Perkin-Elmer Frontier FT-IR instrument as films evaporated from CDCl 3 onto an ATR attachment, where relative intensities are denoted as vw (very weak), w (weak), m (medium), s (strong), and sh (shoulder). All melting points and heat release of neat quadricyclanes were recorded on a Mettler Toledo DSC 2 apparatus. 1 H NMR (400 MHz) and 13 C NMR (100 MHz) spectra were recorded on a Varian 400 MHz instrument or a Bruker 500 MHz instrument with a noninverse cryoprobe using the residual solvent as the internal standard (CDCl 3 , 1 H 7.26 ppm and 13 C 77.16 ppm or d12 -cyclohexane, 1 H 1.38 ppm and 13 C 26.43 ppm). All chemical shifts are quoted on the δ scale (ppm), and all coupling constants (J) are expressed in Hz. All solution-based spectroscopic measurements were performed in cyclohexane in a 1-cm path length cuvette on either a Cary 60 or a Cary 100 UV−Vis spectrophotometer, scanning the wavelength from 600 to 200 nm coupled with Peltier temperature control. Photoswitching for wavelengths 310, 340, 365 and 405 nm were performed using Thorlabs LED lamps M310L3, M340L4, M365F1 and M405LP1 respectively. The thermal back reaction was performed by heating the sample (cuvette) by a Peltier unit in the UV−Vis spectrophotometer. Quantum yields were measured by the published procedure [28] using a high concentration regime (absorption above 2 at the irradiation wavelength) using potassium ferrioxalate and tris-phenanthroline iron (II) complex as a chemical actinometer and Thorlabs LED lamps M310L3, M340L4 and a fiber-coupled LED (M365F1) respectively for irradiation. Irradiation was done perpendicular to the cuvette in a fixed setup approximately 5 cm distance between LED and sample, with stirring, ensuring no movement of the lamp during the experiment. Mass spectra (HRMS) were either acquired by electron spray ionization (ESI) using an Agilent 1260 Infinity fitted with an Agilent 6120 quadrupole for or an ESP-MALDI-FT-ICR spectrometer equipped with a 7 T magnet (calibration of the instrument was done with NaTFA cluster ions). Elemental analyses were performed at London Metropolitan University. Compounds 3 [14] , 12 [27] , and 13 [27] were made by their respective literature methods. Computational methods Calculations for the heat release from QC to NBD were performed at the B3LYP/6-311+G* level  using the NWChem package [30] , [31] . All norbornadiene and quadricyclane compounds were fully relaxed. The storage energy was computed as the energy difference between the norbornadiene and quadricyclane forms. 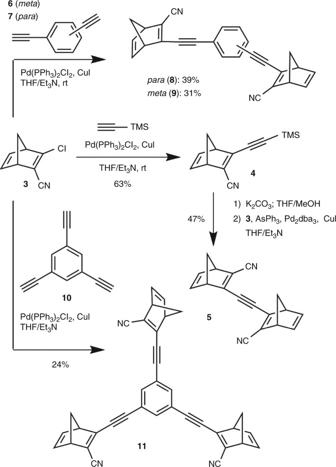Fig. 3 Synthesis of alkyne-linked oligomers. Synthesis of acetylene-linked dimers5,8, and9as well as the trimer11 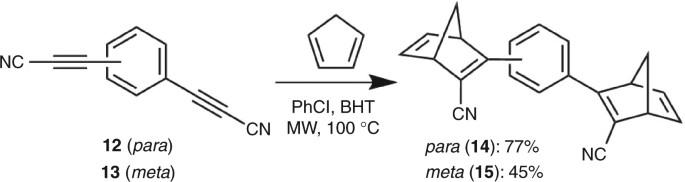Fig. 4 Synthesis of phenylene-linked dimers. Synthesis of phenylene-linked norbornadiene dimers14and15. BHT “butylated hydroxytoluene”, i.e., 2,6-di(tert-butyl)-4-methylphenol; MW microwave heating 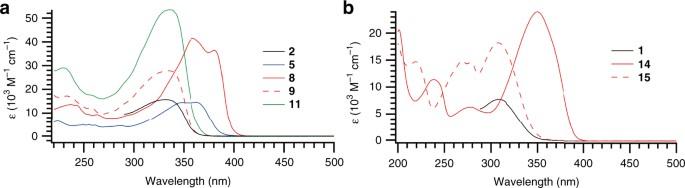Fig. 5 Optical absorption spectra.aUV−Vis absorption spectra of acetylene-linked norbornadienes. Black line:2, blue line:5, red line:8, red dashed line: 9, green line:11.bUV−Vis absorption spectra of phenylene-linked norbornadienes. Black line:1, red line:14, red dashed line:15. The spectra of monomers1and2were recorded in toluene Data availability Data supporting this study can be found in the Supplementary Information file. 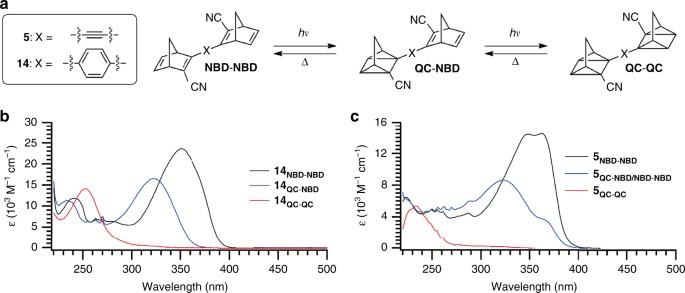Fig. 6 Stepwise conversion of dimers.aStepwise isomerization of5and14to the correspondingQC−NBDandQC−QCisomers.bUV−Vis spectra of14and its isomers. Black line:14NBD−NBD, blue line:14QC−NBD, red line:14QC−QC.cUV−Vis spectra of5,5QC−QCand the thermal-photostationary state between5and5QC−NBD. Black line:5NBD−NBD, blue line: the thermal-photostationary state between5and5QC−NBD, red line:5QC−QC 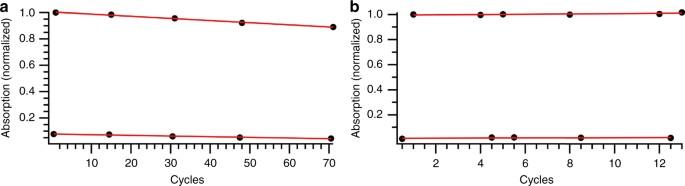Fig. 7 Cyclability test.aCyclability for8showing the normalized absorbance at 362 nm in cyclohexane at 50 °C irradiated at 365 nm.bCyclability for14showing the normalized absorbance at 350 nm in cyclohexane at 70 °C irradiated at 340 nm Upon request to the corresponding author, further information supporting this study can be made available.